Prion-like transmission of neuronal huntingtin aggregates to phagocytic glia in theDrosophilabrain The brain has a limited capacity to self-protect against protein aggregate-associated pathology, and mounting evidence supports a role for phagocytic glia in this process. We have established a Drosophila model to investigate the role of phagocytic glia in clearance of neuronal mutant huntingtin (Htt) aggregates associated with Huntington disease. We find that glia regulate steady-state numbers of Htt aggregates expressed in neurons through a clearance mechanism that requires the glial scavenger receptor Draper and downstream phagocytic engulfment machinery. Remarkably, some of these engulfed neuronal Htt aggregates effect prion-like conversion of soluble, wild-type Htt in the glial cytoplasm. We provide genetic evidence that this conversion depends strictly on the Draper signalling pathway, unveiling a previously unanticipated role for phagocytosis in transfer of pathogenic protein aggregates in an intact brain. These results suggest a potential mechanism by which phagocytic glia contribute to both protein aggregate-related neuroprotection and pathogenesis in neurodegenerative disease. Progressive conversion of normally soluble, cytoplasmic proteins into insoluble, fibrillar, β-sheet-rich aggregates that become sequestered into intracellular inclusion bodies in the central nervous system (CNS) is a robust pathological hallmark of nearly all neurodegenerative disorders, suggesting an intimate connection between abnormal protein homoeostasis and disease pathogenesis [1] . The strong correlation between the spatiotemporal pattern of appearance of these aggregates along neuroanatomical tracts in human Alzheimer disease (AD) and Parkinson disease (PD) brains and the stereotypical patterns of neurological progression of these diseases strongly implicates a role for non-cell-autonomous mechanisms in pathogenesis [2] , [3] . A growing body of evidence supports the hypothesis that physical movement of ordered, fibrillar protein aggregates between cells in the CNS contributes to this propagation by recruiting non-aggregated conformers of the same protein in a process akin to the spread of aggregated PrP Sc in transmissible spongiform encephalopathies and related prion disorders [4] . While both in vitro cell culture studies [5] , [6] , [7] , [8] , [9] , [10] , [11] , [12] , [13] , [14] and in vivo mouse models [11] , [15] , [16] , [17] , [18] , [19] , [20] provide mounting support for a role for prion-like mechanisms in non-cell-autonomous spreading of neurodegenerative diseases, almost nothing is known about the mechanisms by which these agents physically move from one cell to another. The fact that most of the proteins that are recruited into intracellular aggregates associated with neurodegenerative disease pathology normally reside in the cytoplasm presents a cell biological conundrum, because, to propagate from cell to cell, aggregate seeds must find their way from the cytoplasm of a ‘donor’ cell to the cytoplasm of an ‘acceptor’ cell to effect nucleation-driven recruitment of their soluble, cytoplasmic counterparts. While enveloped viruses and some bacterial pathogens have evolved mechanisms that allow them to co-opt membrane trafficking pathways to invade the host cell cytoplasm [21] , [22] , there is no known mechanism by which large, micron-sized fibrillar protein aggregates can travel across the biological membranes. Nonetheless, aggregates of otherwise unrelated disease-associated proteins, including α-synuclein [6] , [14] , huntingtin (Htt) [5] , [8] , [12] , [13] , SOD1 (ref. 9 ), tau [7] , [8] and TDP-43 (ref. 10 ) can be internalized to the cytoplasm of neuronal and nonneuronal acceptor cells in vitro , suggesting that the capacity of aggregates to breach cellular membrane barriers is a widespread cellular property. The possibility that extracellular forms of normally cytoplasmic protein aggregates could be intermediates in the spread of aggregates within the CNS affords potential opportunities for therapeutic interventions specifically targeting these species [23] , [24] and raises the possibility that professional phagocytic glial cells could contribute to either the clearance or dissemination of aggregated species within the brain. Whether protein aggregates directly contribute to neuronal pathogenesis or simply reflect an underlying lesion in protein homoeostasis is not known, but studies in conditional mouse models of neurodegenerative disease reveal that the brain is endowed with the capacity to eliminate aggregates [25] , [26] , and enhancing the pathways responsible for clearance has emerged as a prime therapeutic strategy. Activation of glial phagocytosis is one way by which aggregates or damaged neurons are cleared from the CNS [27] . Microglia and astrocytes respond rapidly to CNS injury by enhanced proliferation, altered morphology and changes in gene expression [28] . While these responses may be initially neuroprotective, prolonged inflammatory responses can become detrimental, and protein aggregation within glia can cause dysfunction that is both intrinsically cytotoxic and negatively influences nearby neurons [29] , [30] , [31] , [32] . Selective silencing of mutant SOD1 expression in microglia significantly delayed disease progression in a mouse model of amyotrophic lateral sclerosis (ALS) [33] , and astrocytes expressing mutant SOD1 or Htt induced toxicity in co-cultured wild-type neurons ex vivo [30] , [31] , [34] , [35] . In this study, we established a Drosophila model to assess the role of phagocytic glia in the uptake and clearance of glutamine-rich (polyQ) aggregates formed by a pathogenic fragment of Htt in neurons within an intact CNS. Huntington disease (HD) is caused by a dominantly inherited mutation that results in the expansion of an N-terminal polyQ tract in Htt above a pathogenic threshold of ∼ 37 glutamines [36] . Htt fragments and fusion proteins containing mutant (polyQ≥37) tracts are highly prone to aggregate into insoluble, fibrillar amyloids in vitro and form cytoplasmic inclusion bodies in vivo [36] . By contrast, Htt fragments containing wild-type (polyQ<37) tracts are soluble, but can be specifically recruited onto seeds consisting of a preformed Htt aggregate [37] , analogous to the conversion of the prion protein PrP C by PrP Sc aggregates [38] . Our data show that mutant Htt aggregates expressed in neurons can be eliminated by glia through a phagocytic process that requires the cell surface engulfment receptor, Draper. Strikingly, we find that phagocytosed neuronal Htt aggregates can access and initiate a prion-like assimilation of normally soluble, wild-type Htt proteins in the glial cell cytoplasm. These findings suggest that phagocytic clearance of neuronal Htt protein aggregates by glia might contribute to the spread of pathogenic protein aggregates in neurodegenerative disease. Clearance of neuronal Htt aggregates by phagocytic glia To assess the clearance of mutant Htt aggregates in the Drosophila brain, we used the QF-QUAS binary expression system [39] to express mutant Htt exon 1 (HttQ91) fused to mCherry fluorescent protein in a single class of olfactory receptor neurons (DA1 ORNs), which have cell bodies in the antenna and project axons that terminate in the DA1 glomerulus of the antennal lobe in the central brain [40] ( Fig. 1a ). Confocal microscopy indicated that HttQ91 expressed in DA1 ORNs was restricted to discrete puncta that were in close proximity to a co-expressed membrane marker, mCD8-green fluorescent protein (GFP), reflecting the high aggregation propensity of this mutant Htt exon 1 fusion protein ( Fig. 1b ). Conversely, mCherry puncta were not detected in DA1 ORNs expressing mCherry-tagged, wild-type Htt exon 1 (HttQ25; Fig. 1b ; Supplementary Fig. 1a,b ). HttQ91 puncta were largely concentrated in the ORN axon terminals in the DA1 glomerulus, where these ORNs synapse with dendrites of projection neurons, and some puncta could also be observed in the DA1 ORN axon bundles along the dorsal surface of the antennal lobe ( Fig. 1c ). The number of HttQ91 puncta reached maximal levels at 1 day after eclosion, and remained constant through adulthood ( Fig. 1d , black bars), suggesting that their rate of formation is balanced by ongoing degradation. 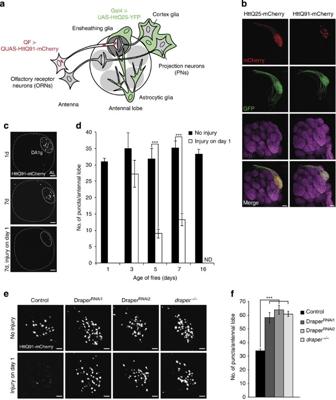Figure 1: HttQ91 aggregates are cleared from ORN axons by phagocytic glia. (a) Cartoon depictingDrosophilaolfactory system circuitry and the glial subtypes present in and around the antennal lobe. To evaluate the fate of HttQ91 aggregates formed in ORNs, a QF driver was used to express HttQ91 in a single class of ORNs whose axons terminate in the DA1 glomerulus of the antennal lobe. To assess transmission of HttQ91 aggregates from ORNs to glia, expression of HttQ91 in DA1 ORNs was coupled with Gal4-mediated expression of HttQ25 in glia. (b) Expression of HttQ25 or HttQ91 in DA1 ORNs. Expression of mCherry-tagged HttQ25 or HttQ91 (red) was restricted to the DA1 glomerulus, indicated by co-expression of the membrane marker mCD8-GFP (green). Antennal lobe neuropil was labelled with antibodies against endogenous Bruchpilot (Brp, magenta). Scale bars, 10 μm. (c) HttQ91 expression in DA1 ORNs without or with antennal injury. Maximum intensity Z-projections of antennal lobes from 1- or 7-day-old adult flies expressing HttQ91 in DA1 ORNs, without or with antennal injury performed on day 1. Boundaries of each antennal lobe (AL; dotted lines) were approximated using DAPI-stained cell body nuclei that mark the periphery of the antennal lobe (not shown), and boundaries of each DA1 glomerulus (DA1g; solid lines) were approximated using HttQ91 signal. Scale bars, 10 μm. (d) Average numbers of HttQ91 aggregates detected in the antennal lobe at the indicated ages without (black bars) or with (white bars) antennal injury were graphed (ND, not determined;n≥10, ±s.e.m., ***P<0.0005, Student’st-test). (e) Draper mediates basal and injury-induced clearance of HttQ91 aggregates from DA1 ORNs. Draper was depleted using two independent UAS-RNAi lines expressed in glia or using thedrprΔ5null mutation (draper−/−), and maximum intensity Z-projections of the DA1 glomerulus from 7-day-old flies without or without antennal injury are shown. Scale bars, 5 μm. (f) Average numbers of HttQ91 puncta were quantified for uninjured 7-day-old adults of the indicated genotype and graphed (n≥8, ±s.e.m., ***P<0.0005, one-way analysis of variance followed by Tukey’spost hoctest). DAPI, 4,6-diamidino-2-phenylindole. Figure 1: HttQ91 aggregates are cleared from ORN axons by phagocytic glia. ( a ) Cartoon depicting Drosophila olfactory system circuitry and the glial subtypes present in and around the antennal lobe. To evaluate the fate of HttQ91 aggregates formed in ORNs, a QF driver was used to express HttQ91 in a single class of ORNs whose axons terminate in the DA1 glomerulus of the antennal lobe. To assess transmission of HttQ91 aggregates from ORNs to glia, expression of HttQ91 in DA1 ORNs was coupled with Gal4-mediated expression of HttQ25 in glia. ( b ) Expression of HttQ25 or HttQ91 in DA1 ORNs. Expression of mCherry-tagged HttQ25 or HttQ91 (red) was restricted to the DA1 glomerulus, indicated by co-expression of the membrane marker mCD8-GFP (green). Antennal lobe neuropil was labelled with antibodies against endogenous Bruchpilot (Brp, magenta). Scale bars, 10 μm. ( c ) HttQ91 expression in DA1 ORNs without or with antennal injury. Maximum intensity Z-projections of antennal lobes from 1- or 7-day-old adult flies expressing HttQ91 in DA1 ORNs, without or with antennal injury performed on day 1. Boundaries of each antennal lobe (AL; dotted lines) were approximated using DAPI-stained cell body nuclei that mark the periphery of the antennal lobe (not shown), and boundaries of each DA1 glomerulus (DA1g; solid lines) were approximated using HttQ91 signal. Scale bars, 10 μm. ( d ) Average numbers of HttQ91 aggregates detected in the antennal lobe at the indicated ages without (black bars) or with (white bars) antennal injury were graphed (ND, not determined; n ≥10, ±s.e.m., *** P <0.0005, Student’s t -test). ( e ) Draper mediates basal and injury-induced clearance of HttQ91 aggregates from DA1 ORNs. Draper was depleted using two independent UAS-RNAi lines expressed in glia or using the drprΔ5 null mutation ( draper −/− ), and maximum intensity Z-projections of the DA1 glomerulus from 7-day-old flies without or without antennal injury are shown. Scale bars, 5 μm. ( f ) Average numbers of HttQ91 puncta were quantified for uninjured 7-day-old adults of the indicated genotype and graphed ( n ≥8, ±s.e.m., *** P <0.0005, one-way analysis of variance followed by Tukey’s post hoc test). DAPI, 4,6-diamidino-2-phenylindole. Full size image To investigate the mechanism by which these aggregates are actively cleared, we performed bilateral antennal axotomy on 1-day-old flies. This injury paradigm has been previously established to induce nearly complete phagocytic clearance of ORN axons undergoing Wallerian degeneration within 5 days [41] . HttQ91 puncta were cleared from the antennal lobe with a similar time-course following injury ( Fig. 1c,d , white bars), suggesting that HttQ91 aggregates and degenerating ORN axons are cleared by a common mechanism. Drosophila phagocytes express a cell surface scavenger receptor, Draper, which initiates an intracellular signalling cascade that promotes engulfment and lysosomal degradation of extracellular debris, such as pruned or damaged axons and dendrites or apoptotic cell corpses [41] , [42] , [43] , [44] , [45] . Draper depletion blocked clearance of HttQ91 aggregates in response to antennal axotomy ( Fig. 1e , bottom row), consistent with Draper’s established role in clearing ORN axonal debris after acute injury [41] . In addition, steady-state numbers of HttQ91 puncta increased nearly twofold in response to depletion of Draper expression using either glial-specific RNA interference (RNAi) or the drprΔ5 null mutation [46] ( Fig. 1e , top row; Fig. 1f ), suggesting that this phagocytic receptor regulates the basal turnover of HttQ91 aggregates in uninjured ORN axons or that it responds to neuronal injury caused by HttQ91 expression. However, we found no evidence for either significantly enhanced ORN axonal membrane loss ( Supplementary Fig. 2a,b ) or activation of the glial JNK ( Supplementary Fig. 3a,b ) and JAK–STAT ( Supplementary Fig. 3c,d ) signalling pathways in response to HttQ91 expression in 7-day-old flies. While we cannot exclude the possibility that HttQ91 expression in DA1 ORNs might cause more subtle neurotoxicity or glial activation, these data suggest that Draper-dependent clearance of HttQ91 aggregates is not accompanied by detectable neuronal degeneration or activation of glial stress signalling. Moreover, Draper depletion caused mCD8-GFP ( Supplementary Fig. 2c,d ) and HttQ91 aggregates ( Fig. 1e,f ) to accumulate in DA1 ORN axons that co-express these two proteins, suggesting that ORN axonal membranes are cleared together with HttQ91 aggregates by Draper-dependent phagocytosis. Therefore, phagocytic glia mediate the turnover of HttQ91 aggregates in axotomized and non-axotomized DA1 ORN axons, suggesting that the same Draper-dependent phagocytic pathway degrades HttQ91 aggregates in response to acute injury or expression of aggregation-prone protein. Prion-like transmission of Htt aggregates from ORNs to glia To test the possibility that phagocytic uptake of HttQ91 aggregates could provide an opportunity for some of these aggregates to gain access to the glial cell cytoplasm, we adapted an assay that we previously established to examine prion-like transmission of Htt aggregates between the cytoplasms of cultured cells [12] , [13] . In this assay, the transfer of mutant Htt aggregates from a ‘donor’ to a ‘recipient’ cell is assessed by monitoring the conversion of wild-type Htt expressed in the cytoplasm of the recipient cell from its normally soluble, diffuse state to an aggregated, punctate form [12] , [13] . Wild-type Htt exon 1 fusion proteins are soluble and lack any organellar or cytoskeletal targeting signals [47] . Consequently, they are diffusely localized throughout the nucleocytoplasmic compartment of cells even upon overexpression. Therefore, the appearance of aggregated, punctate, wild-type Htt necessarily reflects its physical encounter with an aggregated Htt seed in the cytoplasm of the recipient cell. To express Htt exon 1 fusion proteins in glia, we employed the Gal4-UAS binary expression system, which allows for expression of transgenes independently of the QF-QUAS system [39] . HttQ91 expressed using a pan-glial Gal4 driver was present exclusively in puncta throughout glial cell bodies and processes, confirming that HttQ91 aggregation is not a neuron-specific property of HttQ91 in the Drosophila CNS ( Fig. 2a , first column). In contrast, when expressed using the same pan-glial Gal4 driver, HttQ25 was distributed diffusely in the cytoplasm and nucleus of all glia, including those that surround and infiltrate the antennal lobe ( Fig. 2a , second column). However, when HttQ91 and HttQ25 were co-expressed in glia, HttQ25 fluorescence was converted to a punctate pattern that completely co-localized with HttQ91 ( Fig. 2a , third column), demonstrating that aggregated Htt can nucleate the conversion of soluble Htt to an aggregated state when the two proteins co-exist in the same cytoplasm. No such recruitment was observed in flies that express HttQ91-mCherry and GFP lacking a polyQ region ( Fig. 2a , fourth column), confirming that the appearance of green puncta was owing to selective recruitment of polyQ-containing protein and not to global changes in protein solubility. 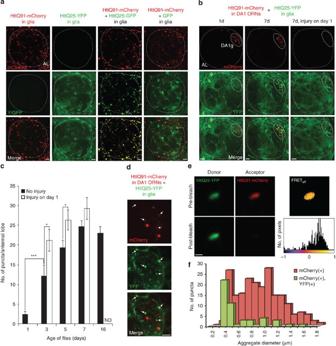Figure 2: Prion-like transfer of HttQ91 aggregates from ORNs to the cytoplasm of glia. (a) HttQ25 aggregates when co-expressed with HttQ91 in glia. Maximum intensity Z-projections of one antennal lobe from 7-day-old adult flies expressing HttQ91-mCherry alone, HttQ25-YFP alone, HttQ91-mCherry and HttQ25-GFP together, or HttQ91-mCherry and GFP together in glia. The approximate boundary of each antennal lobe (‘AL’) is indicated by the dotted lines. Scale bars, 10 μm. (b) Induced aggregation of HttQ25 in glia by expression of HttQ91 in DA1 ORNs. Maximum intensity Z-projections of the antennal lobe from adult flies of the indicated age expressing HttQ91-mCherry in DA1 ORNs and HttQ25-YFP in glia, without or with antennal injury performed on day 1. Approximate boundaries of antennal lobes (AL; dotted line) and DA1 glomeruli (DA1g; solid line) are drawn. Because larger HttQ91 aggregates lacking HttQ25 dominate the red signal, co-localization between HttQ25 and smaller HttQ91 aggregates is underrepresented in the merged images. Seedfor a demonstration of co-localization of HttQ25 with HttQ91 in a single Z-slice. Scale bars, 10 μm. (c) Quantification of glial HttQ25 puncta that were present as the flies aged. The average numbers of HttQ25-YFP puncta detected in each antennal lobe without or with antennal injury were graphed as a function of time (ND, not determined;n≥10, ±s.e.m., *P<0.05, ***P<0.0005, Student’st-test). (d) A single 1.0-μm optical Z-slice from the DA1 glomerulus of a 7-day-old fly with the same genotype as in (b,c). Arrows indicate HttQ25 aggregates (green) that co-localize with HttQ91 signal (red). Scale bar=5 μm. (e) YFP and mCherry fluorescence from a single HttQ25- and HttQ91-containing aggregate before (top) and after (bottom) photobleaching of the mCherry signal. Pixel-by-pixel FRET efficiency is shown in the heat map image and associated histogram. The mean FRET efficiency of the aggregate shown was∼28%. Scale bar, 1 μm. (f) Histogram showing the distribution of diameters for all HttQ91-mCherry puncta detected in the DA1 glomerulus of 7-day-old flies (n=204, red bars), and for those HttQ91-mCherry puncta that co-localized with HttQ25-YFP (green bars). Figure 2: Prion-like transfer of HttQ91 aggregates from ORNs to the cytoplasm of glia. ( a ) HttQ25 aggregates when co-expressed with HttQ91 in glia. Maximum intensity Z-projections of one antennal lobe from 7-day-old adult flies expressing HttQ91-mCherry alone, HttQ25-YFP alone, HttQ91-mCherry and HttQ25-GFP together, or HttQ91-mCherry and GFP together in glia. The approximate boundary of each antennal lobe (‘AL’) is indicated by the dotted lines. Scale bars, 10 μm. ( b ) Induced aggregation of HttQ25 in glia by expression of HttQ91 in DA1 ORNs. Maximum intensity Z-projections of the antennal lobe from adult flies of the indicated age expressing HttQ91-mCherry in DA1 ORNs and HttQ25-YFP in glia, without or with antennal injury performed on day 1. Approximate boundaries of antennal lobes (AL; dotted line) and DA1 glomeruli (DA1g; solid line) are drawn. Because larger HttQ91 aggregates lacking HttQ25 dominate the red signal, co-localization between HttQ25 and smaller HttQ91 aggregates is underrepresented in the merged images. See d for a demonstration of co-localization of HttQ25 with HttQ91 in a single Z-slice. Scale bars, 10 μm. ( c ) Quantification of glial HttQ25 puncta that were present as the flies aged. The average numbers of HttQ25-YFP puncta detected in each antennal lobe without or with antennal injury were graphed as a function of time (ND, not determined; n ≥10, ±s.e.m., * P <0.05, *** P <0.0005, Student’s t -test). ( d ) A single 1.0-μm optical Z-slice from the DA1 glomerulus of a 7-day-old fly with the same genotype as in ( b , c ). Arrows indicate HttQ25 aggregates (green) that co-localize with HttQ91 signal (red). Scale bar=5 μm. ( e ) YFP and mCherry fluorescence from a single HttQ25- and HttQ91-containing aggregate before (top) and after (bottom) photobleaching of the mCherry signal. Pixel-by-pixel FRET efficiency is shown in the heat map image and associated histogram. The mean FRET efficiency of the aggregate shown was ∼ 28%. Scale bar, 1 μm. ( f ) Histogram showing the distribution of diameters for all HttQ91-mCherry puncta detected in the DA1 glomerulus of 7-day-old flies ( n =204, red bars), and for those HttQ91-mCherry puncta that co-localized with HttQ25-YFP (green bars). Full size image To assess the transmission of Htt aggregates from ORNs to glia, we generated double-transgenic flies that simultaneously but independently express mCherry-tagged HttQ91 in DA1 ORNs and yellow fluorescent protein (YFP)-tagged HttQ25 in glia. In 1-day-old flies, HttQ91 fluorescence was punctate, while the HttQ25 signal remained diffuse ( Fig. 2b , first column). However, as the flies aged, HttQ25 puncta could be readily observed, reaching a plateau by 7 days ( Fig. 2b , second column; Fig. 2c, black bars). The majority of these puncta were strongly co-localized with HttQ91 in the DA1 glomerulus and along the dorsal axon bundle. Because HttQ25 does not aggregate when expressed alone in glia ( Fig. 2a , second column), this finding indicates that the presence of aggregated HttQ91 in ORNs markedly influenced the distribution of HttQ25 in neighbouring glia. Importantly, HttQ25 puncta were only detected in glial processes at the DA1 glomerulus, and not in other regions of the antennal lobe, suggesting that close proximity, or possibly direct physical contact between neurons and glia, is required for aggregate transfer. Over 80% of induced YFP-positive HttQ25 puncta in 7-day-old flies strongly co-localized with mCherry-positive HttQ91 puncta ( Fig. 2d , arrows; Supplementary Fig. 4a ), and a fraction of these puncta showed positive fluorescence resonance energy transfer (FRET) signal (mean FRET efficiency=16.34±2.05% s.e.m. ; n =44) between the YFP and mCherry fluorescent protein tags ( Fig. 2e ; Supplementary Fig. 4b ), demonstrating that the two fluorophores are in close molecular proximity (<100 Å). FRET was not detected in puncta that only contained YFP or mCherry signal. Importantly, glial HttQ25 puncta were not detected in flies expressing HttQ25 in DA1 ORNs ( Supplementary Fig. 1a,c ) or in flies that express HttQ91 in DA1 ORNs together with a glial GFP construct lacking the Htt exon 1 polyQ fragment ( Supplementary Fig. 1d ). Thus, HttQ25 aggregation in glia was nucleated by direct physical interaction of cytoplasmic HttQ25 with HttQ91 aggregates that had originated in the cytoplasm of DA1 ORNs. The dependence on detergent solubilization for immunodetection of either HttQ25 or HttQ91 puncta ( Supplementary Fig. 5a,b ) supports the conclusion that neuronal HttQ91 aggregates encountered soluble HttQ25 within a membrane-enclosed compartment and rules out the possibility that this encounter occurred in the extracellular space. HttQ91 aggregates were heterogeneous in size, ranging from ∼ 0.3 to 1.8 μm in diameter ( Fig. 2f , red bars), and, interestingly, those that co-localized with induced HttQ25 puncta in glia ( Fig. 2f , green bars) were distinctly smaller ( ∼ 0.3–0.5 μm), suggesting that smaller Htt aggregates are preferentially transferred from ORNs to glia. Antennal injury enhances ORN-to-glial Htt aggregate transfer To test whether activation of the glial phagocytic response, which promotes the clearance of HttQ91 aggregates from degenerating ORN axons ( Fig. 1e ), also enhances the seeded aggregation of glial HttQ25, we evaluated the distribution of HttQ25 in flies that had undergone bilateral antennal axotomy at 1 day after eclosion ( Fig. 2b,c ). This injury enhanced the formation of HttQ25 puncta in 3- and 5-day-old flies, but had no significant effect at later time points ( Fig. 2c , white bars), consistent with the kinetics of injury-induced ORN axon degeneration previously reported in other models [41] . Therefore, activation of glial phagocytosis enhances both the uptake of neuronal HttQ91 aggregates by glia and the ability of these aggregates to encounter and nucleate conversion of cytoplasmic HttQ25 in glia. Glial Htt aggregates associate with cytoplasmic chaperones Intracellular inclusion bodies into which aggregated proteins such as mutant Htt are deposited are often enriched in cytoplasmic chaperones as well as components of the ubiquitin proteasome system, reflecting the view that these diseases are strongly linked to perturbed protein homoeostasis [48] . Indeed, we found that both HttQ91 and HttQ25 puncta were robustly ( ∼ 50–73%) labelled with antibodies to the endogenous cytoplasmic chaperones, Hsp70/Hsc70 and Hsp90 ( Fig. 3a,b,d , red and green bars), in flies expressing HttQ91 in DA1 ORNs and HttQ25 in glia. Likewise, ∼ 36% and ∼ 51% of HttQ25 puncta that co-localized with HttQ91 were labelled with Hsp70/Hsc70 and Hsp90 antibodies ( Fig. 3d , yellow bars), respectively, consistent with our observation that ∼ 80% of total HttQ25 puncta were associated with a visible HttQ91 seed ( Fig. 2d ; Supplementary Fig. 4a ). The strong association with these cytoplasmic chaperones supports the conclusion that Htt aggregates in both ORNs and glia have access to the cytoplasmic compartment. Surprisingly, antibodies against endogenous ubiquitin robustly ( ∼ 61%) labelled HttQ91 aggregates, but not HttQ25 aggregates or the smaller HttQ91 puncta with which they are co-localized ( ∼ 4%; Fig. 3c,d ). This observation supports the conclusion that at least two populations of HttQ91 aggregates exist: smaller, ubiquitin-negative puncta that are preferentially transferred to glia, and larger, ubiquitin-positive puncta that do not co-localize with glial HttQ25. This polymorphism among HttQ91 aggregates in the Drosophila CNS echoes previous observations that Htt aggregation in cell culture [49] and mouse [50] models of HD is processive and that ubiquitin is recruited only to larger, mature aggregates. 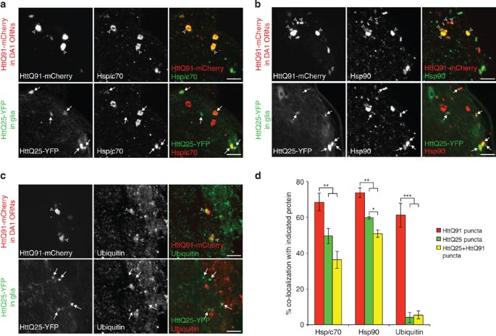Figure 3: Neuronal HttQ91 and glial HttQ25 aggregates associate with cytoplasmic markers. (a–c) Co-localization of HttQ91 or HttQ25 aggregates with the endogenous cytoplasmic markers Hsp70/Hsc70, Hsp90 and ubiquitin. Single 1.0-μm optical Z-slices from the DA1 glomerulus of 7-day-old adult flies expressing HttQ91-mCherry in DA1 ORNs and HttQ25-YFP in glia and immunostained with antibodies against Hsp70/Hsc70 (a), Hsp90 (b) and ubiquitin (c) are shown. Unfilled arrowheads indicate HttQ91 aggregates that lack associated HttQ25 signal, and filled arrows indicate induced HttQ25 aggregates in glia. Scale bars, 5 μm. (d) Quantification of the % co-localization of each aggregate subtype with the endogenous cytoplasmic markers (n≥4, ±s.e.m., *P<0.05, **P<0.01, ***P<0.001, one-way analysis of variance followed by Tukey’spost hoctest). Figure 3: Neuronal HttQ91 and glial HttQ25 aggregates associate with cytoplasmic markers. ( a – c ) Co-localization of HttQ91 or HttQ25 aggregates with the endogenous cytoplasmic markers Hsp70/Hsc70, Hsp90 and ubiquitin. Single 1.0-μm optical Z-slices from the DA1 glomerulus of 7-day-old adult flies expressing HttQ91-mCherry in DA1 ORNs and HttQ25-YFP in glia and immunostained with antibodies against Hsp70/Hsc70 ( a ), Hsp90 ( b ) and ubiquitin ( c ) are shown. Unfilled arrowheads indicate HttQ91 aggregates that lack associated HttQ25 signal, and filled arrows indicate induced HttQ25 aggregates in glia. Scale bars, 5 μm. ( d ) Quantification of the % co-localization of each aggregate subtype with the endogenous cytoplasmic markers ( n ≥4, ±s.e.m., * P <0.05, ** P <0.01, *** P <0.001, one-way analysis of variance followed by Tukey’s post hoc test). Full size image ORN-to-glia Htt aggregate transfer requires Draper signalling The finding that Draper is essential for clearance of HttQ91 aggregates from axotomized or non-axotomized ORN axons ( Fig. 1e,f ) led us to consider whether Draper is also required for transmission of these aggregates from ORNs to the glial cytoplasm. To test for a role of Draper in this process, we depleted Draper expression using glial-specific RNAi or the drprΔ5 null mutation in flies expressing HttQ91 in DA1 ORNs and HttQ25 in glia. Loss of Draper expression by either method completely inhibited the formation of glial HttQ25 aggregates in uninjured animals ( Fig. 4a,b ). Thus, non-injury-induced, Draper-dependent phagocytic uptake of ORN-derived Htt aggregates is essential not only for clearance but also for HttQ91 aggregates to access the glial cytoplasm where they can nucleate wild-type HttQ25 aggregation. 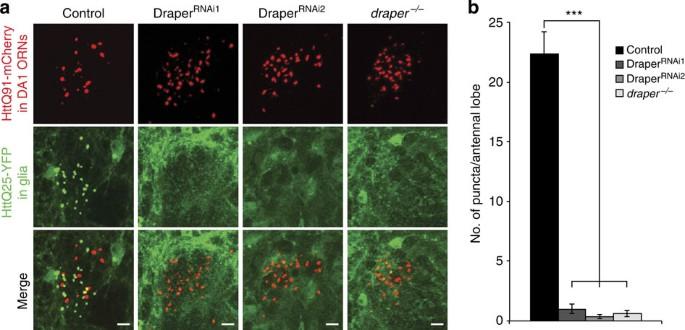Figure 4: Draper is required for nucleation of glial HttQ25 aggregation by neuronal HttQ91 aggregates. (a) Draper is essential for transfer of HttQ91 aggregates from DA1 ORN axons to the glial cytoplasm. Maximum intensity Z-projections of the DA1 glomerulus from 7-day-old adult fly brains expressing HttQ91-mCherry in DA1 ORNs and HttQ25-YFP in glia, either without (control) or with depletion of Draper expression using two independent RNAi lines (DraperRNAi1and DraperRNAi2) or thedrprΔ5null mutation (draper−/−). Scale bars, 5 μm. (b) Quantification of the number of induced HttQ25 aggregates detected in the antennal lobe of 7-day-old adult flies as ina(n≥8, ±s.e.m., ***P<0.0005, one-way analysis of variance followed by Tukey’spost hoctest). Figure 4: Draper is required for nucleation of glial HttQ25 aggregation by neuronal HttQ91 aggregates. ( a ) Draper is essential for transfer of HttQ91 aggregates from DA1 ORN axons to the glial cytoplasm. Maximum intensity Z-projections of the DA1 glomerulus from 7-day-old adult fly brains expressing HttQ91-mCherry in DA1 ORNs and HttQ25-YFP in glia, either without (control) or with depletion of Draper expression using two independent RNAi lines (Draper RNAi1 and Draper RNAi2 ) or the drprΔ5 null mutation ( draper −/− ). Scale bars, 5 μm. ( b ) Quantification of the number of induced HttQ25 aggregates detected in the antennal lobe of 7-day-old adult flies as in a ( n ≥8, ±s.e.m., *** P <0.0005, one-way analysis of variance followed by Tukey’s post hoc test). Full size image Activation of Draper-dependent phagocytosis requires phosphorylation of the intracellular domain of Draper and consequent binding of the non-receptor tyrosine kinase, shark, to these phosphorylated sites [51] . Like Draper, shark is essential for recruitment of glial membranes to injured ORN axons and subsequent engulfment and degradation of debris. To test whether shark also mediates the basal clearance of HttQ91 aggregates and/or their entry into the glial cytoplasm in a similar manner to Draper, we used an RNAi line previously shown to block the clearance of ORN axonal debris formed after antennal injury [51] . Knockdown of shark in 7-day-old animals increased the steady-state levels of HttQ91 puncta in uninjured ORN axons ( Fig. 5a,b,j ) and inhibited HttQ91 aggregate clearance from severed ORN axons ( Supplementary Fig. 6a,b ) to the same extent as that observed after Draper depletion. Shark knockdown also abolished the formation of HttQ25 aggregates in glia ( Fig. 5a,b,k ), demonstrating that Draper–shark signalling is essential for the transfer of HttQ91 aggregates from ORNs to the glial cytoplasm. 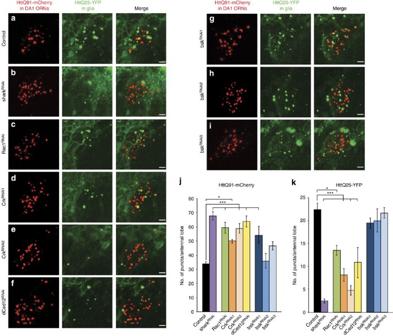Figure 5: Nucleation of glial HttQ25 aggregation by neuronal HttQ91 aggregates requires phagocytic engulfment genes. (a–k) Shark, Rac1, Crk and dCed12 mediate entry of HttQ91 aggregates into the glial cytoplasm to induce aggregation of HttQ25. Maximum intensity Z-projections of the DA1 glomerulus from 6- to 8-day-old adult fly brains expressing HttQ91-mCherry in DA1 ORNs and HttQ25-YFP in glia, without (a) or with (b–i) glial expression of double-stranded RNAs targeting shark (b), Rac1 (c), Crk (d,e), dCed12 (f) or bsk (g–i). Scale bars, 5 μm. (j,k) Average numbers of HttQ91 aggregates (j) or induced HttQ25 aggregates (k) detected in the antennal lobe of 6– to 8-day-old adult fly brains as shown ina–i(n≥8, ±s.e.m., *P<0.05, **P<0.005, ***P<0.0005, one-way analysis of variance followed by Tukey’spost hoctest). Figure 5: Nucleation of glial HttQ25 aggregation by neuronal HttQ91 aggregates requires phagocytic engulfment genes. ( a – k ) Shark, Rac1, Crk and dCed12 mediate entry of HttQ91 aggregates into the glial cytoplasm to induce aggregation of HttQ25. Maximum intensity Z-projections of the DA1 glomerulus from 6- to 8-day-old adult fly brains expressing HttQ91-mCherry in DA1 ORNs and HttQ25-YFP in glia, without ( a ) or with ( b – i ) glial expression of double-stranded RNAs targeting shark ( b ), Rac1 ( c ), Crk ( d , e ), dCed12 ( f ) or bsk ( g – i ). Scale bars, 5 μm. ( j , k ) Average numbers of HttQ91 aggregates ( j ) or induced HttQ25 aggregates ( k ) detected in the antennal lobe of 6– to 8-day-old adult fly brains as shown in a – i ( n ≥8, ±s.e.m., * P <0.05, ** P <0.005, *** P <0.0005, one-way analysis of variance followed by Tukey’s post hoc test). Full size image The small GTPase Rac1 regulates cytoskeletal rearrangement during phagocytic events [52] . In Drosophila , glial Rac1 and a guanine nucleotide exchange factor complex formed by the proteins Crk, Mbc and dCed12 mediate the engulfment of ORN axonal debris targeted by activated Draper [53] . Knockdown of Rac1, Crk or dCed12 inhibited basal and injury-induced clearance of HttQ91 aggregates from DA1 ORN axons ( Fig. 5c–f,j ; Supplementary Fig. 6c–f ) and the formation of HttQ25 aggregates in glia ( Fig. 5c–f,k ), suggesting that Rac1 and the Crk/Mbc/dCed12 guanine nucleotide exchange factor complex are required for the entry of neuronal HttQ91 aggregates into the glial cytoplasm. Basket (bsk), the Drosophila ortholog of c-Jun kinase, upregulates Draper gene expression in response to antennal ablation through a MAP kinase signalling pathway and is required for the extension of glial membranes to engulfment targets in the antennal lobe [54] . Surprisingly, bsk knockdown did not result in a significant impairment of HttQ25 puncta formation ( Fig. 5g–i,k ), even though all three bsk RNAi lines strongly inhibited injury-induced HttQ91 aggregate clearance ( Supplementary Fig. 6g–i ). Therefore, bsk is required for the injury-induced clearance of degenerating ORN axons, but is dispensable for the ability of these neuronal aggregates to enter the glial cytoplasm and nucleate the aggregation of soluble HttQ25. In this study, we have established a Drosophila model that demonstrates an essential role for phagocytic glia in clearance of Htt aggregates from ORN axons undergoing Wallerian degeneration after antennal axotomy or from non-severed axons. Our data show that HttQ91 aggregate clearance is mediated by a pathway that requires the glial engulfment receptor Draper and downstream genes, and is genetically indistinguishable from the pathway that operates in other glial phagocytic processes, including clearance of axonal or cellular debris following injury and axon pruning during development. Surprisingly, we find that HttQ91 aggregates taken up by this Draper-dependent process are able to access and initiate a prion-like conversion of normally soluble, cytoplasmic HttQ25 in glia. These two findings have important implications for the potential role of glia in the suppression and/or progression of neurodegenerative diseases. Glial phagocytosis plays an important neuroprotective role in response to many types of brain injury, including insults associated with the production of neurodegenerative disease-linked insoluble protein aggregates [27] , [28] . Secretion of pro-inflammatory cytokines and opsonins by activated glia promotes phagocytic clearance of damaged neurons, neuronal processes and cellular debris [27] , [55] . In vitro , mouse astrocytes can bind to and degrade extracellular Aβ aggregates in cell culture and in brain slices [56] . In vivo , pharmacological activation of microglia promotes clearance of Aβ deposits in a transgenic mouse model of AD [57] , and antibodies against Aβ or α-synuclein promote microglial-mediated phagocytic removal of the corresponding extracellular aggregates [58] , [59] . Compelling evidence for a neuroprotective role for glial phagocytosis has come from recent studies linking missense mutations in TREM2, which encodes a microglial phagocytic receptor, to several neurodegenerative diseases including AD, PD and ALS [60] , [61] , [62] , [63] . Our data establish an essential role for phagocytic glia in clearance of HttQ91 aggregates from ORN axons, but whether this phagocytosis is initiated as a specific response to the presence of aggregates or a collateral result of constitutive axon turnover and remodelling is unclear. This strict dependence on phagocytosis contrasts with previous work showing that extracellular aggregates can enter the cytoplasms of many different types of cultured cells, and cell surface proteins are only partially responsible for this entry [7] , [8] , [9] , [12] , [13] . It is likely that the discrepancy between these previous studies and the current one at least in part reflects differences in the extracellular environment in cell culture, which is homogeneous and effectively infinite, and in the intact brain, where extracellular space is severely restricted in volume and is continuously patrolled by phagocytic glia. This view is supported by our observations that, in the fly brain, aggregate uptake by glia occurred only in close proximity to ORN axons containing HttQ91 aggregates and that detergent solubilization was required to immunolabel the aggregates. We therefore favour a mechanism in which HttQ91 aggregates are phagocytosed by glia together with surrounding axonal membrane, analogous to the process by which supernumerary synapses are eliminated by Draper in Drosophila development [64] and by the mammalian Draper orthologue, MEGF10, in the adult mouse brain [65] . Our observation that phagocytosed neuronal HttQ91 aggregates can nucleate aggregation of cytoplasmic HttQ25 in glia is surprising because phagocytosis normally leads to encapsulation and degradation of internalized debris within the membrane-enclosed phagolysosomal system. However, our study provides two independent lines of evidence to support the conclusion that ORN-derived HttQ91 aggregates encounter HttQ25 in the glial cytoplasm. First, because HttQ25 is a highly soluble protein that does not aggregate in cells unless seeded by a pre-existing aggregate, the strict dependence of HttQ25 puncta formation on HttQ91 expression in ORNs indicates that these two Htt species must have physically interacted with one another. In principle, it is possible that, instead of HttQ91 aggregates being internalized by glia, this transfer could occur in the opposite direction, namely by the transfer of soluble HttQ25 into ORNs. However, the finding that HttQ25 aggregation was blocked by glial-specific knockdown of Draper and enhanced by antennal injury indicates an absolute requirement for phagocytic uptake of HttQ91, supporting ORN-to-glia transfer. Second, the majority of HttQ91 and HttQ25 aggregates co-localize with the cytoplasmic chaperones Hsp70/Hsc70 and Hsp90, indicating that aggregated HttQ25 is in direct contact with the cytoplasm. It is conceivable that merging of the phagocytic and autophaghic pathways could provide an opportunity for HttQ91 aggregates and soluble HttQ25 to encounter one another. However, we failed to detect substantial (<15%) co-localization of either HttQ91 or HttQ25 puncta with the autophagy markers, Atg8 and p62, or with the early endosome marker, Rab5 (data not shown). Moreover, the amount of soluble HttQ25 that could be captured within an autophagosome is miniscule compared with the total cytoplasmic pool that would be available to be nucleated by an internalized HttQ91 seed. Altogether, these data strongly support the conclusion that phagocytosed HttQ91 aggregates are able to access the glial cytoplasm, thereby affording the opportunity to effect prion-like spreading of disease pathology. How do these engulfed HttQ91 aggregates breach the membrane barrier that separates the phagolysosomal lumen from the cytoplasm? The dependence of this process on Draper, shark and the actin-remodelling complex indicates that aggregates must access the glial cytoplasm at a step during or subsequent to phagocytic engulfment. It is possible that cytoplasmic entry could be facilitated by interference of phagocytosed aggregates with membrane fusion events during phagosome maturation. However, this ‘foot-in-the-door’ mechanism would be favoured by larger aggregates, which is in opposition to our finding that smaller HttQ91 aggregates are more strongly associated with cytoplasmic nucleation of glial HttQ25. We propose instead that slow or inefficient completion of membrane fusion events could provide a temporary conduit to the cytoplasm for HttQ91 aggregates. Such a mechanism would predict an upper size limit for cytoplasmic entry that could be exploited by small, newly formed aggregates. This prediction is supported by our finding that the neither the induced HttQ25 aggregates nor the co-localized nucleating HttQ91 puncta in glia are labelled with antibodies to ubiquitin, a marker previously identified with more mature, larger Htt puncta in both cell culture [49] and transgenic mouse [50] models of HD. The findings described here have broader implications for how potentially toxic protein aggregates are dispersed throughout the diseased brains. Phagocytic removal of aggregates is neuroprotective, but it is likely that phagocytes become impaired in their ability to clear debris as disease worsens and that chronic glial activation becomes detrimental to the health of nearby neurons. Our finding that phagocytosed neuronal Htt aggregates can enter the glial cytoplasm suggests that this transfer process could generate a reservoir of prion-like species inside glia, possibly facilitating their spread to other cells. A growing body of evidence supports the view that glial dysfunction exacerbates neurodegenerative disease pathogenesis by influencing the survival of neurons [66] , and determining the mechanism(s) by which glia contribute to toxicity will be of great value to the development of therapeutic strategies to combat these devastating disorders. Fly husbandry Drosophila stocks were maintained on a standard cornmeal/sugar/agar medium at 22 °C, and matings were performed at 25 °C. The repo-Gal4 (M1B) and Or67d-QF drivers were used to express transgenes in all glia and DA1 ORNs, which expresses the odorant receptor Or67d, respectively. Other transgenic and RNAi lines that were not generated in this study include QUAS-mCD8-GFP [39] , UAS-drprRNAi#5A (‘Draper RNAi1 ’), UAS-drprRNAi#3b (‘Draper RNAi2 ’), UAS-shark RNAi#6b (refs 41 , 51 ; kind gifts from M. Freeman, UMass Medical School), UAS-Rac1 RNAi#49247 , UAS-Crk RNAi#19061 (‘Crk RNAi1 ’), UAS-Crk RNAi#106498 (‘Crk RNAi2 ’), UAS-dCed12 RNAi#10455 , UAS-bsk RNAi#18155 (‘bsk RNAi1 ’), UAS-bsk RNAi#34138 (‘bsk RNAi2 ’), UAS-bsk RNAi#34139 (‘bsk RNAi3 ’; Vienna Drosophila Resource Center), TRE-GFP [67] and 10xStat92E-GFP [68] . Flies containing the drprΔ5 null mutation [41] were a kind gift from M. Freeman, UMass Medical School. Fly genotypes used in each figure are listed in Supplementary Table 1 . Cloning and transgenesis Htt exon 1 transgenes containing CAG repeat region lengths of either 25 (wild-type) or 91 (mutant) and fused at the C-terminus to GFP, YFP or mCherry fluorescent protein were PCR amplified from pcDNA3.1 mammalian expression plasmids [13] and inserted into the pUASTattB Drosophila expression plasmid downstream of a 5XUAS sequence to allow for Gal4-driven expression. These transgenes plus the attB bacterial attachment site region of pUASTattB were further subcloned into the pQUAST plasmid [39] . Transgenic lines containing fluorescent protein-tagged UAS- or QUAS-Htt exon 1 transgenes were generated by φC31-mediated site-specific integration into the attP3 (X) or attP24 (II) docking sites [69] . Integration of each transgene was confirmed by PCR analysis of genomic DNA isolated from single males. Expression of each UAS or QUAS transgene was tested by crossing the flies with a Gal4 or QF driver, respectively, and imaging fixed brains by confocal microscopy (see below). Brain dissection, immunostaining and imaging Adult fly brains were dissected, fixed and stained using standard dissection procedures. Briefly, brains were dissected into ice-cold PBS/T (PBS containing either 0.01% Triton X-100 when intrinsic fluorescence of the GFP, YFP or mCherry fusions was to be examined, or 0.1% Triton X-100 when immunostaining was to be performed). The brains were transferred to microfuge tubes containing PBS/T+4% paraformaldehyde and fixed while rocking at room temperature in the dark for 20 min. Brains were washed with PBS/T for 2 × 1, 1 × 5 and 3 × 20 min at room temperature in the dark. For examining intrinsic fluorescence, the brains were then stained with PBS/0.01%T containing 250 ng ml −1 DAPI (Life Technologies) for 30 min at room temperature in the dark, followed by 2 × 1- and 1 × 15-min washes. For immunostaining, the brains were blocked in PBS/0.1%T containing 5% normal goat serum (Lampire Biological Products) for 30 min at room temperature, followed by incubation in primary antibodies diluted in blocking buffer overnight at 4 °C. The brains were washed in PBS/0.1%T for 2 × 1, 1 × 5, 3 × 20 min and 1 × 1 h at room temperature, followed by incubation in secondary antibodies diluted in blocking buffer overnight at 4 °C, washing in PBS/0.1%T for 2 × 1, 1 × 5, 3 × 20 min and 1–2 × 1 h, incubating in PBS/0.1%T containing 250 ng ml −1 DAPI (Invitrogen) for 30 min in the dark, and finally washing in PBS/0.1%T for 2 × 1 and 1 × 15 min at room temperature. After the final wash, any remaining liquid was removed from the brains and replaced with Slowfade Gold Antifade Reagent (Life Technologies). Brains were incubated for 1h to overnight at 4 °C in the dark, and then bridge-mounted on glass microscope slides in Slowfade reagent before imaging on a Zeiss LSM 510 or 780 laser scanning microscope equipped with 40X and 63X, 1.4 numerical aperture oil objectives to obtain optical z-slices. Primary antibodies were used at the following dilutions: chicken anti-GFP (1:1,000; Aves Labs; number GFP-1020), rabbit anti-GFP (1:4,000; Molecular Probes; number A6455), rabbit anti-DsRed (1:2,000; Clontech; number 632496), mouse anti-Bruchpilot (1:50; Developmental Studies Hybridoma Bank; number nc82), mouse anti-hsp70/hsc70 clone BB70 (1:100; Enzo Life Sciences; number ADI-SPA-822), rat anti-hsp90 clone 16F1 (1:100; Enzo Life Sciences; number ADI-SPA-835) and mouse anti-ubiquitin (clone FK2; 1:250; BioMol; number Cay14220). Secondary antibodies and dilutions used were: FITC anti-chicken (1:500; Jackson Immunoresearch Laboratories, Inc.; number 703-095-155), Cy3 anti-rabbit (1:1,000; Jackson Immunoresearch Laboratories, Inc.; number 111-165-003) and Alexa Fluor 647 anti-rabbit or anti-mouse (1:250; Life Technologies; numbers A-21244 or A-21235). Aggregate quantification To quantify HttQ91-mCherry puncta, images were rendered in three dimensions using Imaris imaging software (Bitplane), and the Spots Region Growing algorithm was selected to count non-uniformly sized objects. The largely diffuse expression of HttQ25-YFP in glia generated a high background signal that made use of image analysis software to detect individual induced HttQ25 puncta at the DA1 glomerulus impractical, so we instead manually scored HttQ25-YFP puncta by analysing contiguous optical z-slices through each antennal lobe. Scoring was independently performed by two investigators who were blind to the experimental conditions. Fluorescence intensity quantification mCD8-GFP fluorescence was quantified by measuring the fluorescence intensity of a 7.44 × 7.44 × 5-μm 3 cube positioned in the centre of a sum-intensity Z-stack of the DA1 glomerulus. Fluorescence of the TRE-GFP or 10xStat92E-GFP reporters was quantified by measuring the fluorescence intensity of three different regions of interest at standardized positions in or around the antennal lobe. All image analyses were performed using ImageJ software (NIH). FRET measurements by acceptor photobleaching FRET between YFP and mCherry fluorescent protein tags on HttQ25 and HttQ91, respectively, was measured by monitoring dequenching of YFP donor fluorescence after photobleaching of mCherry acceptor (using a 561-nm laser set at 100% intensity) on a Leica SP5 confocal microscope equipped with a 63X, 1.4 numerical aperture oil objective. HttQ25/HttQ91 co-localized puncta were selected for FRET analysis to have sufficient mCherry signal to enable detection of YFP dequenching after mCherry photobleaching. YFP fluorescence was excited using a 514-nm laser and emission detected between 525 and 555 nm, and mCherry was excited with a 561-nm laser and emission collected between 610 and 675 nm; with these settings, no bleedthrough between the channels was observed. FRET efficiencies (FRET eff ) for individual puncta were calculated after background correction by subtracting donor fluorescence intensity before acceptor photobleaching (YFP initial ) from donor fluorescence intensity after bleaching (YFP final ), dividing this value by YFP final and multiplying by 100. All fluorescence intensity measurements were performed using ImageJ software (NIH). The pixel-by-pixel FRET eff image in Fig. 2e was generated using the AccPbFRET plug-in for ImageJ [70] . Statistics Quantified data presented all figures are shown as mean±s.e.m. The number of subjects is indicated by n , and was selected to yield sufficient statistical power. Statistical analyses were performed using one-way analysis of variance followed by Tukey’s post hoc test or using unpaired, two-tailed Student’s t -test, as indicated in the Figure legends. How to cite this article: Pearce, M. M. P. et al . Prion-like transmission of neuronal huntingtin aggregates to phagocytic glia in the Drosophila brain. Nat. Commun . 6:6768 doi: 10.1038/ncomms7768 (2015).